Single-vesicle architecture of synaptobrevin2 in astrocytes Exocytic transmitter release is regulated by the SNARE complex, which contains a vesicular protein, synaptobrevin2 (Sb2). However, Sb2 vesicular arrangement is unclear. Here we use super-resolution fluorescence microscopy to study the prevalence and distribution of endogenous and exogenous Sb2 in single vesicles of astrocytes, the most abundant glial cells in the brain. We tag Sb2 protein at C- and N termini with a pair of fluorophores, which allows us to determine the Sb2 length and geometry. To estimate total number of Sb2 proteins per vesicle and the quantity necessary for the formation of fusion pores, we treat cells with ATP to stimulate Ca 2+ -dependent exocytosis, increase intracellular alkalinity to enhance the fluorescence presentation of yellow-shifted pHluorin (YpH), appended to the vesicle lumen domain of Sb2, and perform photobleaching of YpH fluorophores. Fluorescence intensity analysis reveals that the total number of endogenous Sb2 units or molecules per vesicle is ≤25. Astrocytes provide metabolic support to neurons, actively tune synaptic activity and influence the microcirculation of the brain [1] . A key process mediating astrocyte communication with neighbouring cells is regulated exocytosis. This multi-stage, spatially and temporally highly organized process consists of many steps leading to merger between secretory organelles and the plasma membrane. Astrocytic secretory organelles may contain gliotransmitters (peptides, amino acids and/or nucleotides), membrane transporters, channels and/or other signalling molecules [2] , [3] . Distinct secretory organelle types [4] , [5] , [6] can be engaged in regulated exocytosis [7] and they are differentially regulated. Vesicular exocytosis is mediated by Sb2 (ref. 8 ), also referred to as VAMP2, while lysosomal exocytosis is thought to be governed by VAMP7 (ref. 9 ). Thus, to understand the nature of the exocytotic process and its role in astrocyte communication, one needs to understand secretory organelle architecture at the highest possible spatial resolution in living cells. Individual vesicles can be studied by labelling proteins that allow the vesicular fusion process. Therefore, one can mark Sb2, which is typically present on the vesicle membrane in astrocytes [10] , [11] . Our knowledge regarding the architecture of biological organelles and their function at the cellular and subcellular level in living cells arises mainly from studies using microscopic techniques, such as confocal laser scanning microscopy (CLSM) [12] , [13] . However, the resolution limit of CLSM, dictated by diffraction [14] , impedes the ability to study single-cell organelles smaller than the limit of transverse and axial resolution (~200 nm and ~500 nm, respectively). This limit can be overcome by super-resolution microscope techniques [15] , which include structured illumination microscopy (SIM) with improved transverse resolution to ~100 nm [16] , thus allowing punctiform object measurements at the nanoscale level. Furthermore, as exploited in the present work, SIM can also report on inter-fluorophore distances at a fraction of its resolution limit. To study how Sb2 is structurally integrated and distributed in single vesicles, we examined the arrangement of this vesicle membrane protein in fixed and living cultured astrocytes. As a dimensional calibration, we measured the length between two fluorescent tags placed at two ends of a Sb2 protein at the single-vesicle level. Analysis of the intensity of fluorescent tags, reporting on the number of molecules, revealed a multimodal distribution with equally interspaced peaks. We conclude that there are ≤25 molecules of endogenous Sb2 per vesicle in astrocytes. Arrangement of Sb2 on a single vesicle To describe the structural integration of Sb2 proteins in a single vesicle at the nanometer scale, we designed a genetically modified protein chimera, yellow synaptopHluorin (YSpH) with yellow-shifted superecliptic pHluorin (YpH; a derivative of pHluorin [17] , a modified enhanced green fluorescent protein (EGFP)) targeted to the vesicle lumen (labelled as A in Fig. 1a ), by attaching it to the C terminus of Sb2 via an 8-amino-acid (aa) linker ( Supplementary Fig. 1a ). The N-terminus of the same protein was marked with an anti-Sb2 antibody (recognizing aa 1–18 of rat Sb2), which was tagged with secondary antibodies conjugated with Atto 594, a rhodamine derivative dye, that has excitation and emission wavelengths spectrally compatible with YpH (labelled as B in Fig. 1a ). By considering the length of the Sb2 protein to be 46 nm in its elongated or uncoiled form [18] , [19] , [20] , [21] and the average length of an IgG antibody molecule (between 11.5 nm and 14 nm for two different configurations) [22] , we predicted a structural arrangement as shown in Fig. 1a . As controls, we made additional genetically encoded Sb2 constructs. To avoid the use of antibodies, we fused YSpH with red fluorescent protein (mCherry) on the cytoplasmic vesicle side (that is, N-terminus) of Sb2 (mCherry-YSpH) ( Supplementary Fig. 2 ). In this construct, inter-fluorophore (centre-centre) distance of ~54 nm is predicted, where one considers an average aa residue size of 0.4 nm (ref. 20 ) (thus, for the full length of 116 aa of Sb2 along with 8 aa of the linker, there is total of 124 aa × 0.4 nm=49.6 nm) and EGFP size of 4.7 nm [23] along with an assumption of a similar size for mCherry. It should be noted that for YSpH construct decorated with the primary antibody against Sb2 and Atto-labelled secondary antibody, the YpH-Atto inter-fluorophore distance is predicted to be ~75–80 nm (assuming a linear arrangement of two antibody molecules in shorter and longer configurations, respectively, as well as a negligible size of Atto in comparison with EGFP). We also prepared another chimeric protein (YSpH-7aa-mCherry) ( Supplementary Fig. 2 ) that had mCherry attached, via a 7-aa residue linker (~2.8 nm), to C terminus of YpH, with a predicted inter-fluorophore distance up to ~7.5 nm. 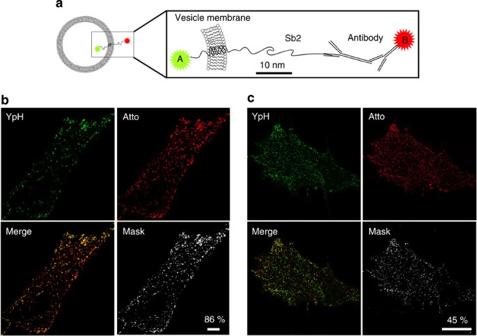Figure 1: Vesicle-associated membrane protein Sb2 fluorescently labelled at the luminal and cytoplasmic sides of the vesicle membrane. (a) The diagram represents an astrocytic vesicle (left) in which a version of Sb2 is expressed, with a fluorescent protein in the vesicle lumen (fluorophore A, that is, YpH) and with an immunolabelled cytoplasmic domain (fluorophore B, that is, Atto 594). The boxed diagram on right shows the architecture of Sb2 across the vesicle membrane, drawn to scale by considering the length of Sb218,19.bandcare images from CLSM and SIM, respectively. To stain Sb2 in vesicle lumen, astrocytes were transfected with a plasmid encoding YSpH (green). To stain the N-terminal part of Sb2 located on the cytosolic side of the vesicle membrane, primary antibody against Sb2 and a secondary antibody conjugated to Atto 594 (Atto; red) were used. Merge panels show overlay of YSpH and Atto signals arising from the vesicle lumen and the cytoplasm. Mask panels show only the colocalized pixels between YpH and Atto. Bar, 10 μm. Note the smaller amount of colocalization (percent, shown for representative single astrocytes) in the SIM image than in the CLSM image. Figure 1: Vesicle-associated membrane protein Sb2 fluorescently labelled at the luminal and cytoplasmic sides of the vesicle membrane. ( a ) The diagram represents an astrocytic vesicle (left) in which a version of Sb2 is expressed, with a fluorescent protein in the vesicle lumen (fluorophore A, that is, YpH) and with an immunolabelled cytoplasmic domain (fluorophore B, that is, Atto 594). The boxed diagram on right shows the architecture of Sb2 across the vesicle membrane, drawn to scale by considering the length of Sb2 [18] , [19] . b and c are images from CLSM and SIM, respectively. To stain Sb2 in vesicle lumen, astrocytes were transfected with a plasmid encoding YSpH (green). To stain the N-terminal part of Sb2 located on the cytosolic side of the vesicle membrane, primary antibody against Sb2 and a secondary antibody conjugated to Atto 594 (Atto; red) were used. Merge panels show overlay of YSpH and Atto signals arising from the vesicle lumen and the cytoplasm. Mask panels show only the colocalized pixels between YpH and Atto. Bar, 10 μm. Note the smaller amount of colocalization (percent, shown for representative single astrocytes) in the SIM image than in the CLSM image. Full size image We transfected astrocytes with a plasmid encoding YSpH (shown in green on images, YpH) and subsequently exposed these cells to immunocytochemical labelling with primary antibodies against Sb2 followed by fluorescently tagged secondary antibodies (Atto 594; shown in red in Fig. 1a ). Antibody binds to exogenously expressed Sb2, that is, YpH, as well as its endogenous nonfluorescent form. As shown in Fig. 1 , we determined the degree of colocalization (%) between YpH and antibody-conjugated Atto, which significantly differed ( P <0.001; Student’s t -test) when obtained by CLSM (83±2%, n =20 cells) and SIM (40±4%, n =9 cells). The reduced colocalization in SIM images is consistent with the idea that YpH and Atto fluorophores, associated with imaged structures or vesicles, are present in close proximity, not overlapping completely [24] . To verify this notion, we further studied individual fluorescent puncta, representing single vesicles. Chemical fixation (see Methods) of the cells enhanced YpH signal due to pH equilibration between vesicles and the extracellular medium. Pairs of YpH and Atto SIM signals exhibit different patterns ( Fig. 2a–d ). After eliminating YpH and Atto signals that were >200 nm apart from each other (15–20% of the puncta), four pattern categories, in descending preponderance, were observed: (a) partial overlapping YpH and Atto signals ( Fig. 2a ); (b) partial overlapping YpH and Atto signals, as in pattern (a), but the average Atto signal exhibited higher intensity than the YpH signal ( Fig. 2b ); (c) overlapping YpH and Atto signals ( Fig. 2c ); and (d) Atto enveloped YpH signal, which in cross-sectional fluorescence profiles may appear as a YpH signal sandwiched between two Atto signals ( Fig. 2d ). The proportions of these patterns were as follows: for (a) 44±2%; (b) 34±2%; (c) 15±3%; and (d) 7±1% ( n =349 vesicles, 3 cells) ( Fig. 2e ). All arrangements were further studied by plotting normalized intensity line profiles for each of these arrangements ( Fig. 2 , mid column), which were used to measure the distance between peaks of Gaussian curves, fitted to the intensity of YpH and Atto signals. The frequency distribution plot for the distance, measured in each pair of YpH and Atto fluorophores, yielded a mean value of 65±2 nm ( n =541, 5 cells) ( Fig. 2f ). The measured distance, when compared with predicted values (75–80 nm), could represent an underestimate if the orientation of Sb2 and associated antibodies are not parallel to the focal plane and/or if their configurations are not so ‘linear’ as indicated in Fig. 1a (that is, antibodies assume angles and Sb2 coils). 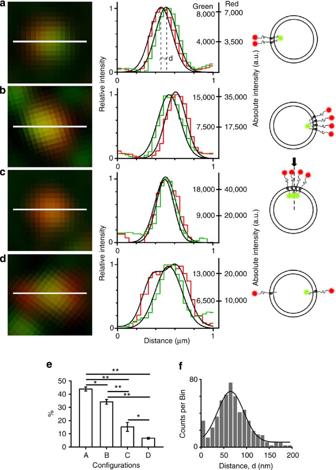Figure 2: Patterns of two Sb2-associated fluorophores reveal nonuniform vesicular distribution of Sb2. (a–d) Each panel contains (left to right) a SIM image, a graph and a drawing. SIM images (left column) show different patterns of Atto (red) and YpH (green) fluorophores tagging Sb2. Graphs (middle column) show normalized/relative fluorescence intensity profiles (red and green fluorescence along the section, that is, line, in corresponding SIM image). The right ordinates of the intensity profiles show absolute intensity (a.u., arbitrary unit) of green and red fluorescent puncta. Schematics in the right column show possible arrangements of two fluorophores in a single vesicle. The arrow and vertical dash-line are drawn to visualize the top view of the fluorophore pair (c). The order of images (a–d) is according to abundance (shown in %) of the pattern observed in astrocytes as summarized in graph (e). The error bars represent s.e.m. We analyzed three astrocytes in which a total of 349 vesicles were examined. *P<0.02 and **P<0.001 (ANOVA). As indicated in line profile ina, distance (proximity) between the green and red fluorophores,d, can be determined as the distance between the peaks. The frequency distribution plot of inter-fluorophore distance measured for all YpH-Atto pairs is shown inf. The mean value for the distance between YpH and Atto is 65±2 nm (mean±s.e.m.), which is calculated by fitting a Gaussian curve (f) on a frequency distribution plot of the form Counts/bin={A/[σ(✓2π)]} × exp{−[x−μ)2/2σ2]} (Equation 1) where x=distance (nm), total countA=(4,295±503);σ=28.6; μ=(65±2) nm. The squared correlation coefficientR2=0.90,n=541 vesicles, 5 cells; difference from zero was statistically significant (P<0.001; ANOVA). Figure 2: Patterns of two Sb2-associated fluorophores reveal nonuniform vesicular distribution of Sb2. ( a – d ) Each panel contains (left to right) a SIM image, a graph and a drawing. SIM images (left column) show different patterns of Atto (red) and YpH (green) fluorophores tagging Sb2. Graphs (middle column) show normalized/relative fluorescence intensity profiles (red and green fluorescence along the section, that is, line, in corresponding SIM image). The right ordinates of the intensity profiles show absolute intensity (a.u., arbitrary unit) of green and red fluorescent puncta. Schematics in the right column show possible arrangements of two fluorophores in a single vesicle. The arrow and vertical dash-line are drawn to visualize the top view of the fluorophore pair ( c ). The order of images ( a – d ) is according to abundance (shown in %) of the pattern observed in astrocytes as summarized in graph ( e ). The error bars represent s.e.m. We analyzed three astrocytes in which a total of 349 vesicles were examined. * P <0.02 and ** P <0.001 (ANOVA). As indicated in line profile in a , distance (proximity) between the green and red fluorophores, d , can be determined as the distance between the peaks. The frequency distribution plot of inter-fluorophore distance measured for all YpH-Atto pairs is shown in f . The mean value for the distance between YpH and Atto is 65±2 nm (mean±s.e.m. ), which is calculated by fitting a Gaussian curve ( f ) on a frequency distribution plot of the form Counts/bin={ A /[ σ ( ✓ 2π)]} × exp{−[x−μ) 2 /2 σ 2 ]} (Equation 1) where x=distance (nm), total count A =(4,295±503); σ =28.6; μ=(65±2) nm. The squared correlation coefficient R 2 =0.90, n =541 vesicles, 5 cells; difference from zero was statistically significant ( P <0.001; ANOVA). Full size image To further verify that this measurement of inter-fluorophore distance is associated with the distance between C- and N termini of Sb2 across the vesicle membrane, we transfected astrocytes to express mCherry-YSpH, an additional Sb2 construct ( Supplementary Fig. 2 ), having red fluorescent protein (mCherry) appended to the N terminus (located at the vesicular cytosolic side) of YSpH; YpH at the C terminus is located in the vesicular lumen. The results revealed a mean inter-fluorophore (mCherry-YpH) distance of 57±1 nm ( n =403 vesicles, 7 cells; Fig. 3d ), which is in good agreement with the predicted inter-fluorophore distance (54 nm) in this Sb2 chimera, but significantly different ( P =0.004; analysis of variance (ANOVA) from YpH-Atto measurements in Fig. 2f . This difference can likely be attributed to the length of attached antibodies when studying YpH-Atto pairs. It cannot be ruled out that the mCherry-YpH measurements may represent the distance between fluorophores of two different Sb2 molecules located on adjacent vesicles, although this scenario is unlikely. As an additional cross-check measure, we expressed a chimeric protein with mCherry appended via a 7-aa linker to C terminus of YpH (YSpH-7aa-mCherry) ( Supplementary Fig. 2 ) and recorded an inter-fluorophore distance of 0±5 nm ( n =338 vesicles, 6 cells; Fig. 3h ), a measurement that is consistent with the predicted value (7.5 nm). 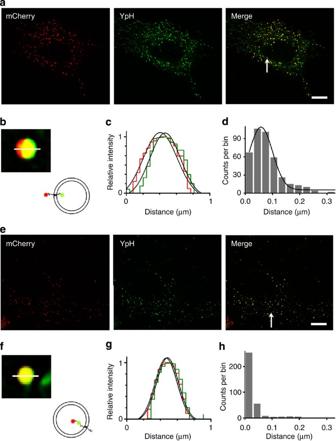Figure 3: SIM measurements of the distance between fluorescent proteins appended to Sb2 termini. aandeare the SIM images showing astrocytes transfected with mCherry-YSpH and YSpH-7aa-mCherry plasmids, respectively. Bar, 10 μm. Merge panels show the overlay of the fluorescence of mCherry (red) and YpH (green) signals.bandfare close-up images of the mCherry and YpH pairs obtained from the images (Merge, arrow) inaande, respectively. The inset drawings indicate the orientation of YpH and mCherry decorating Sb2.candgshow relative fluorescence intensity profiles along the lines drawn inbandf. The histogramsdandhshow frequency distribution plots of the distances between the two fluorophores. (d) In case of mCherry-YSpH, the mean value of the distance (peak-to-peak, as inFig. 2a) between YpH (intravesicular) and mCherry (cytoplasmic) is 57±1 nm (mean±s.e.m.) (R2=0.98,n=403 vesicles, 7 cells; significantly different than zero,P<0.001; ANOVA). To measure the peak-to-peak distance, we fitted Gaussian curves using Equation 1. (h) In the case of YSpH-7aa-mCherry, the mean distance between two fluorophores juxta-positioned (spacing provided by a 7-aa linker) in the vesicular lumen is negligible (0±5 nm;n=338 vesicles, 6 cells). Figure 3: SIM measurements of the distance between fluorescent proteins appended to Sb2 termini. a and e are the SIM images showing astrocytes transfected with mCherry-YSpH and YSpH-7aa-mCherry plasmids, respectively. Bar, 10 μm. Merge panels show the overlay of the fluorescence of mCherry (red) and YpH (green) signals. b and f are close-up images of the mCherry and YpH pairs obtained from the images (Merge, arrow) in a and e , respectively. The inset drawings indicate the orientation of YpH and mCherry decorating Sb2. c and g show relative fluorescence intensity profiles along the lines drawn in b and f . The histograms d and h show frequency distribution plots of the distances between the two fluorophores. ( d ) In case of mCherry-YSpH, the mean value of the distance (peak-to-peak, as in Fig. 2a ) between YpH (intravesicular) and mCherry (cytoplasmic) is 57±1 nm (mean±s.e.m.) ( R 2 =0.98, n =403 vesicles, 7 cells; significantly different than zero, P <0.001; ANOVA). To measure the peak-to-peak distance, we fitted Gaussian curves using Equation 1. ( h ) In the case of YSpH-7aa-mCherry, the mean distance between two fluorophores juxta-positioned (spacing provided by a 7-aa linker) in the vesicular lumen is negligible (0±5 nm; n =338 vesicles, 6 cells). Full size image Diameter measurements of pHluorin-laden vesicles We next assessed vesicular diameter using an approach involving filling the vesicle lumen in live astrocytes using LysoTracker Red DND-99, which stains acidic organelles within a cell [25] . The specificity of monitoring secretory vesicles was obtained by transfecting astrocytes to express YSpH and hence label Sb2-positive vesicles, before their exposure to LysoTracker. Subsequently, we analysed only dually, YSpH and LysoTracker, labelled puncta or vesicles ( Fig. 4a,b ) by obtaining Gaussian curves of the intensity profiles along a line section through the equatorial plane of such vesicles ( Fig. 4c ). The YSpH Gaussian curves of individual puncta were narrower and eccentrically positioned when compared with those of matching individual LysoTracker puncta, indicating that YSpH is non-uniformly distributed and does not completely disclose vesicular lumen ( Fig. 4c ). Nonetheless, by measuring the full width at half maximum intensity (FWHM) of the Gaussian curve of red LysoTracker fluorescence ( Fig. 4c,d ), we determined the apparent diameter of astrocytic vesicles of 305±3 nm ( n =129 vesicles, 9 cells). It should be noted that this estimate of the vesicle diameter, which is in reasonable agreement with the previously obtained measurements or Sb2-laden vesicles in live astrocytes [26] , is based on only a fraction of LysoTracker-positive vesicles in which YpH signal is significant, due to either a relatively high copy number of YSpH molecules and/or a relatively more alkaline vesicle lumen. In addition, LysoTracker-based measurement may overestimate vesicular diameter, as is the case when measuring the diameter of standard fluorescent beads (nominally 200 nm in diameter with measured FWHM of ~255 nm, Supplementary Fig. 3c ). Nonetheless, the Sb2-laden vesicles that we have interrogated in live astrocytes have an apparent size of ~300 nm in diameter. 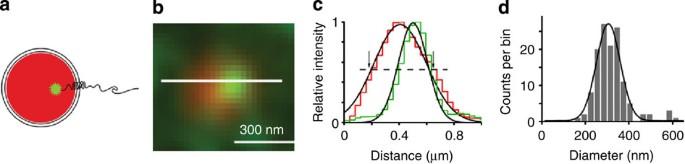Figure 4: Measurement of vesicle diameter in live astrocytes by SIM. (a) Diagram of an astrocytic vesicle loaded with LysoTracker DND-99 (red), expressing YSpH (green) and (b) the corresponding SIM image in a live astrocyte. Bar, 300 nm. (c) Fluorescence intensity profile of LysoTracker and YpH in the vesicle lumen along the line drawn inb. The dashed line indicates how the apparent diameter of a vesicle was determined, by measuring the FWHM of Gaussian curve of the red fluorophore. Note the intersection with Gaussian curve drawn on normalized intensity of the red fluorophore, marked with arrows. (d) The frequency distribution plot for apparent vesicle diameter, as defined inc. The mean value (mean±s.e.m.) of the apparent vesicle diameter is 305±3 nm (n=129 vesicles, 9 cells), measured by fitting a Gaussian curve of the form described in Equation 1 (R2=0.94; significantly different from zero,P<0.001; ANOVA). Figure 4: Measurement of vesicle diameter in live astrocytes by SIM. ( a ) Diagram of an astrocytic vesicle loaded with LysoTracker DND-99 (red), expressing YSpH (green) and ( b ) the corresponding SIM image in a live astrocyte. Bar, 300 nm. ( c ) Fluorescence intensity profile of LysoTracker and YpH in the vesicle lumen along the line drawn in b . The dashed line indicates how the apparent diameter of a vesicle was determined, by measuring the FWHM of Gaussian curve of the red fluorophore. Note the intersection with Gaussian curve drawn on normalized intensity of the red fluorophore, marked with arrows. ( d ) The frequency distribution plot for apparent vesicle diameter, as defined in c . The mean value (mean±s.e.m.) of the apparent vesicle diameter is 305±3 nm ( n =129 vesicles, 9 cells), measured by fitting a Gaussian curve of the form described in Equation 1 ( R 2 =0.94; significantly different from zero, P <0.001; ANOVA). Full size image The number of exogenous Sb2 molecules on single vesicles To learn about the putative number of Sb2 molecules per vesicle or fluorescent punctum, we initially made a comparative analysis of the intensities of fluorophores that were used to label Sb2 and of those obtained from standard, dye-loaded spherical latex particles, that is, green fluorescent beads ( Supplementary Fig. 3 ). Close inspection of the frequency histograms of fluorescence intensities of beads ( Supplementary Fig. 3d ) and fluorophore-tagged Sb2 (YpH, Supplementary Fig. 3e ; Atto, Supplementary Fig. 3f ) revealed that the distribution of bead and YpH intensity values exhibit single-mode distributions ( Supplementary Fig. 3d,e , respectively), albeit YpH, unlike bead fluorescence, is skewed from normality (D’Agostino test P <0.01 and P >0.05, respectively). Of note, each distribution here contains signals from many puncta (for comparison with individual YSpH punctum see Fig. 4b ). It should be noted that the YpH labelling only discloses a subset of vesicles containing exogenous Sb2, that is, YSpH. However, when all (endogenous and exogenous) Sb2 molecules are labelled using antibodies, there are apparent multiple modes in the Atto intensities frequency histogram ( Supplementary Fig. 3f ). Although this optical fluorescence intensity method does not distinguish single molecules from other unitary or quantal intensities (a finite fluorescence ‘packet’), these results are consistent with the notion that Sb2 is non-uniformly distributed and that likely there is on average more than one unit or molecule of Sb2 present on the surface of a single vesicle, which we investigated further below. Of course, a fluorescent bead contains more than one molecule of dye, but as the dye loading is uniform throughout the bead as per its amorphous polymer backbone, the bead population fluorescence intensity distribution shows an appearance of a single ‘packet’. In YSpH-expressing astrocytes that were immunolabelled by an anti-Sb2 antibody conjugated with Atto dye, we did not observe a correlation between the fluorescence intensity and the area of the Atto fluorescent puncta ( R 2 =0.05, P =0.28). In an attempt to determine the approximate number of Sb2 molecules laden in each vesicle and used in the process of vesicular fusion, using CLSM, we have monitored vesicle YSpH fluorescence in live astrocytes that were stimulated by ATP (0.1 mM). By activating purinergic receptors, ATP increases cytosolic Ca 2+ and promotes the merger between the vesicle and the plasma membrane, leading to the formation of a fusion pore [12] , [26] , [27] , [28] . On fusion pore formation, alkalinization of the vesicle lumen is expected, as vesicular protons exit into the extracellular medium. This would be reflected by an increase in YSpH fluorescence emission. Alternatively, the vesicular lumen can be chemically alkalinized, so that, even when the fusion pore is closed, YSpH signal increases ( Supplementary Fig. 1c,d ). Full alkalinization of vesicles can be accomplished by the application of NH 4 Cl [29] , [30] . Hence, to assess the extent to which ATP stimulation (with the main conduit for protons to exit the vesicle lumen via Ca 2+ -dependent fusion pore opening) elicited vesicle alkalinization, we subsequently added NH 4 Cl (45 mM) to the bath to increase vesicle lumen pH independent of the fusion pore formation ( Fig. 5a ). It should be noted that inherent to our experimental design, here we could only interrogate those vesicles that undergo kiss and run with stable pore formation of varying duration (see below), but not the full fusions, where the vesicle collapses into the plasma membrane. 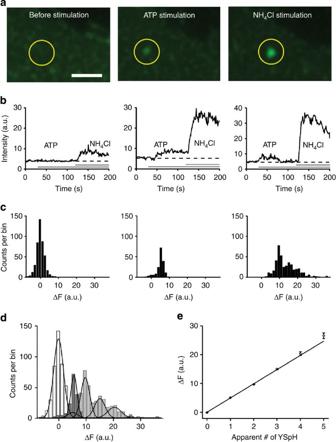Figure 5: Stimulation of YSpH-labelled vesicles by ATP and NH4Cl reveals the number of YSpH molecules present on a single astrocytic vesicle. (a) Time series frames of a representative YSpH-positive vesicle (circle) recorded by CLSM before and after successive stimulations with ATP and NH4Cl. Bar, 1 μm. (b) Examples of time-dependent changes in the fluorescence intensity of individual vesicles: left panel, ATP failed to evoke an increase in fluorescence intensity, however, NH4Cl elicited an increase; middle panel, application of ATP elicited a sustained increase in fluorescence intensity that was augmented by NH4Cl; and right panel, ATP elicited a transient increase in fluorescence intensity, which was followed with NH4Cl-elicited increase. Horizontal grey bars indicate the timing of ATP/NH4Cl applications. (c) Amplitude distributions of the change in YSpH fluorescence intensity (ΔF) recorded in nine astrocytes before and after stimulations (bin width=1.5 a.u.). Left panel, the change in YSpH intensity plot represents a background, which was obtained by monitoring changes in YSpH intensity before and after addition (at 30 s for 10 s) of ATP (bottom horizontal line) in recordings where ATP failed to elicit a significant increase in YSpH. Middle panel, after ATP, and, right panel, subsequent NH4Cl applications, the intensity distribution incrementally shifts to the right as vesicles alkalinize due to the pore formation (ATP) and subsequent chemical alkalinization (NH4Cl), respectively. (d) Combined plot of the change in YSpH intensity distributions for all vesicles (n=1,045) from nine astrocytes: background (white) and after stimulation with ATP (dark grey) and NH4Cl (light grey). The Gaussian curves are fitted by keeping the s.d. as determined in the background shown in left panel and using Equation 1 (where x=ΔF (a.u.), for fitting parameters seeTable 1). (e) The peaks of the Gaussian fits of different modes of intensities (obtained ind) are plotted as a function of modes, that is, number of YSpH packets; the relationship can be described using a liner regression in the form: ΔF (a.u.)=(4.95±0.04) × apparent # of YSpH+(−0.02±0.05), where # is the number or multiples of YSpH molecules (R2=0.997; significantly different from zero,P<0.001; ANOVA). Figure 5: Stimulation of YSpH-labelled vesicles by ATP and NH 4 Cl reveals the number of YSpH molecules present on a single astrocytic vesicle. ( a ) Time series frames of a representative YSpH-positive vesicle (circle) recorded by CLSM before and after successive stimulations with ATP and NH 4 Cl. Bar, 1 μm. ( b ) Examples of time-dependent changes in the fluorescence intensity of individual vesicles: left panel, ATP failed to evoke an increase in fluorescence intensity, however, NH 4 Cl elicited an increase; middle panel, application of ATP elicited a sustained increase in fluorescence intensity that was augmented by NH 4 Cl; and right panel, ATP elicited a transient increase in fluorescence intensity, which was followed with NH 4 Cl-elicited increase. Horizontal grey bars indicate the timing of ATP/NH 4 Cl applications. ( c ) Amplitude distributions of the change in YSpH fluorescence intensity (ΔF) recorded in nine astrocytes before and after stimulations (bin width=1.5 a.u.). Left panel, the change in YSpH intensity plot represents a background, which was obtained by monitoring changes in YSpH intensity before and after addition (at 30 s for 10 s) of ATP (bottom horizontal line) in recordings where ATP failed to elicit a significant increase in YSpH. Middle panel, after ATP, and, right panel, subsequent NH 4 Cl applications, the intensity distribution incrementally shifts to the right as vesicles alkalinize due to the pore formation (ATP) and subsequent chemical alkalinization (NH 4 Cl), respectively. ( d ) Combined plot of the change in YSpH intensity distributions for all vesicles ( n =1,045) from nine astrocytes: background (white) and after stimulation with ATP (dark grey) and NH 4 Cl (light grey). The Gaussian curves are fitted by keeping the s.d. as determined in the background shown in left panel and using Equation 1 (where x=ΔF (a.u. ), for fitting parameters see Table 1 ). ( e ) The peaks of the Gaussian fits of different modes of intensities (obtained in d ) are plotted as a function of modes, that is, number of YSpH packets; the relationship can be described using a liner regression in the form: ΔF (a.u. )=(4.95±0.04) × apparent # of YSpH+(−0.02±0.05), where # is the number or multiples of YSpH molecules ( R 2 =0.997; significantly different from zero, P <0.001; ANOVA). Full size image The individual vesicles of astrocytes subjected to the above experimental paradigm show three types of responses ( Fig. 5b ): (i) ATP stimulation failed to increase YSpH fluorescence, whereas the ensuing application of NH 4 Cl increased YSpH fluorescence (to reveal the presence of chimeric Sb2), which was the most abundant pattern occurring in ~60% of cases (261 of 430 vesicles; 9 cells) and likely representing failure of fusion pore opening ( Fig. 5b , left); (ii) ATP caused a persistent increase in YSpH fluorescence intensity, which was further increased by the subsequent addition of NH 4 Cl, a response occurring in ~35% ( n =149 vesicles; 9 cells) of cases ( Fig. 5a and b , middle) and (iii) ATP evoked a transient increase in YSpH fluorescence intensity, which returned to resting levels before the increase in YSpH fluorescence intensity was elicited by NH 4 Cl, an outcome occurring in ~5% ( n =20 vesicles; 9 cells) of all cases ( Fig. 5b , right). The latter two ATP-productive types of responses (ii and iii) likely represent cases where ATP stimulation was associated with a fusion pore opening, which was either persistently open, throughout the time-course of our approach, in the former case (ii), or opened only transiently in the latter case (iii). Such fusion pore changes have been described in astrocytes [26] and in other cell types [31] , [32] . Next, we used the change in YSpH intensity measurements from individual vesicles obtained in the above described experiments to generate YSpH intensity distributions at resting (no vesicular fusions)/background condition, as well as during the sequential stimulation with ATP and NH 4 Cl. Our aim was to define the putative number of YSpH (that is, exogenous Sb2) molecules in fusion pore forming single vesicles. We first obtained the distribution of the noise (basal level of YSpH) intensity changes, which expectedly yielded an average fluorescence change near zero ( Fig. 5c , left). We then obtained distributions of YSpH intensity changes during productive ATP stimulation ( Fig. 5c , middle) and subsequent chemical alkalinization of vesicles with NH 4 Cl ( Fig. 5c , right). All distributions were fitted with Gaussian curves using Equation 1 (with x=ΔF; see fitting parameters in Table 1 ) to obtain multimodal values for all the distributions ( Fig. 5d ). As one would expect, the first mode corresponds to background YSpH intensity changes ( Fig. 5d , open bars), while the second mode represents the quantum of YSpH intensity change due to the stimulation, with subsequent modes being integer multiples. Surprisingly, ATP stimulation generated only one mode, that of the single quantum ( Fig. 5c , middle and Figure 5d , dark grey), while NH 4 Cl, beside the single quantum, also generated integer multiples ( Fig. 5c , right and Fig. 5d , light grey). This implicates a differential accessibility of vesicular lumen to de-protonation of YpH fluorophore during physiological ATP stimulation, as opposed to enforced chemical alkalinization by NH 4 Cl (see Discussion). Nonetheless, these modal peaks of YSpH fluorescence are distributed as multiples of fundamental quantal unit, likely representing the number of YSpH molecules within individual vesicles, as revealed by a linear relationship between the apparent number of YSpH molecules and change in YSpH intensity ( Fig. 5e ). Our results indicate that there are maximum of five units or molecules of YSpH, that is, exogenous Sb2, in an astrocytic vesicle. However, only one YSpH molecule appeared necessary for fusion pore formation as per ATP stimulation data. Table 1 Area under curve ( A ) and mean value of each peak ( μ ) obtained from Gaussian curves in stimulation experiment. Full size table Photobleaching of YpH authenticates the number of exogenous Sb2 molecules We performed photobleaching experiments to cross-check the above determined number of YSpH molecules in a single vesicle. As above, we transfected the astrocytes to express YSpH and stimulated them with NH 4 Cl solution. The CLSM imaging was accomplished using regular (as above) laser power and detector gain settings. The bleaching of YpH fluorophores was done by increasing the laser power by the factor of 2–3. We observed two types of YpH fluorescence decay: (a) apparent exponential and (b) stepwise decays occurring in ~30% and ~70%, respectively, out of total analyzed events ( n =277). We selected the stepwise events to analyse the number of YSpH molecules. We observed different step decreases in YSpH fluorescence intensity originating from individual vesicles. 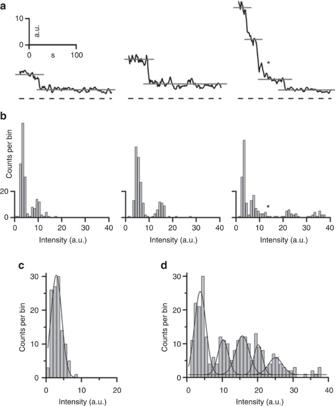Figure 6: Photobleaching of NH4Cl-alkalinized YSpH-laden vesicles confirms the number of YSpH molecules present on a single astrocytic vesicle. (a) Examples of time-dependent changes in the fluorescence intensity signals of individual vesicles: left panel, a single step decrease in the YpH fluorescence, middle panel, a single step decrease in the YpH fluorescence with double amplitude, compared with the event shown in the left panel, and, right panel, multiple step decreases in YpH fluorescence with three discrete steps, ‘*’ denotes another step decrease, which according to frequency plot does not represent a discrete step, but rather belongs to the distribution of the final discrete step. Dashed lines represent the baseline (zero-line) and grey lines show the levels of YpH fluorescence signals at discrete steps. (b) The respective distributions of the fluorescence intensity amplitudes of signals shown in the panela. The first peak in amplitude plots denotes the lowest intensity observed. (c) The intensity distribution of the background, which was obtained by measuring the fluorescence intensity of the vesicle surroundings after 180 s of bleaching (R2=0.95;n=108 events; bin width=1.5 a.u.). (d) Fluorescence intensity distribution of YSpH-labelled vesicles after bleaching (R2=0.91;n=277 vesicles; bin width=1.5 a.u.). The Gaussian curves are fitted by using Equation 1 (x=Intensity (a.u.); see fitting parameters inTable 2). Figure 6a displays three representative examples of such events: (i) a small step decrease in YpH fluorescence, (ii) a step decrease by the factor of two, compared with the former event and (iii) an event with three discrete step decreases in YpH fluorescence ( Fig. 6a ). By plotting the frequency distribution of the above type of events ( Fig. 6b ), we observed distinct modes of YSpH fluorescence intensity. The background intensity in this set of experiments was measured in near vicinity of vesicles ( n =108 events). The distribution of the background fluorescence could be fitted by a Gaussian curve (Equation 1, where x=Intensity (a.u. ); R 2 =0.95, see fitting parameters in Table 2 ) and yielded distribution with the mean value of 2.9±0.1 a.u (mean±s.e.m., Fig. 6c ). Similarly, we obtained the distribution of the YSpH intensity changes due to photobleaching of NH 4 Cl alkalinized vesicles, which showed multi-modality ( Fig. 6d ; R 2 =0.91, see fitting parameters in Table 2 ). As one would expect, the first mode corresponds to background YSpH intensity changes, while the remaining four equidistant modes, report on the discrete intensities (that is, quanta), corresponding to the number of YSpH molecules in a single vesicle of live astrocytes ( Fig. 6d ; compared with Fig. 5d ). This number of YSpH molecules obtained from photobleaching experiments validates the quantification obtained using the YSpH increase in fluorescence due to ATP and NH 4 Cl stimulation ( Fig. 5e ). We further analyzed exponential decays of the bleaching events of YSpH. The average time constant ( τ ) is ~30 s ( n =14 vesicles), which means that on average it takes 30 s to bleach 63% of the total number of Sb2 molecules present on a vesicle, that is, three YSpH molecules bleach out of total five in 30 s. Therefore, it is likely (more than 10% probability) that two YSpH will bleach simultaneously, especially following the start of the bleaching procedure. In agreement, the percentage of events with the double amplitude ( Fig. 6a , middle) of the total bleaching events was 16.6%. Figure 6: Photobleaching of NH 4 Cl-alkalinized YSpH-laden vesicles confirms the number of YSpH molecules present on a single astrocytic vesicle. ( a ) Examples of time-dependent changes in the fluorescence intensity signals of individual vesicles: left panel, a single step decrease in the YpH fluorescence, middle panel, a single step decrease in the YpH fluorescence with double amplitude, compared with the event shown in the left panel, and, right panel, multiple step decreases in YpH fluorescence with three discrete steps, ‘*’ denotes another step decrease, which according to frequency plot does not represent a discrete step, but rather belongs to the distribution of the final discrete step. Dashed lines represent the baseline (zero-line) and grey lines show the levels of YpH fluorescence signals at discrete steps. ( b ) The respective distributions of the fluorescence intensity amplitudes of signals shown in the panel a . The first peak in amplitude plots denotes the lowest intensity observed. ( c ) The intensity distribution of the background, which was obtained by measuring the fluorescence intensity of the vesicle surroundings after 180 s of bleaching ( R 2 =0.95; n =108 events; bin width=1.5 a.u.). ( d ) Fluorescence intensity distribution of YSpH-labelled vesicles after bleaching ( R 2 =0.91; n =277 vesicles; bin width=1.5 a.u.). The Gaussian curves are fitted by using Equation 1 (x=Intensity (a.u. ); see fitting parameters in Table 2 ). Full size image Table 2 Area under curve ( A ) and mean value of each peak ( μ ) obtained from Gaussian curves in bleaching experiment. Full size table The ratio between exogenous and endogenous Sb2 molecules To obtain the number of endogenous Sb2 molecules present on individual astrocytic vesicles, we used Sb2 immunolabelling of astrocytes transfected to express YSpH. Such individual astrocytes contain a mixture of vesicles, those laden with endogenous Sb2 alone (Atto positive, YpH negative) along with others that are dually laden with both endogenous Sb2 and YSpH (Atto and YpH positive) ( Fig. 7a left). In addition, we compared the Sb2 immunoreactivity Atto signals of dually laden vesicles to those of native vesicles from untransfected astrocytes ( Fig. 7a right). The distributions and cumulative plots of Atto fluorescence intensity of Sb2-immunolabelled vesicles that besides endogenous Sb2 (w/o YSpH; n =262) contain exogenous Sb2 in form of YSpH (w YSpH; n =958) show larger median values for Atto signals ( Fig. 7b ); the additional fluorescence of vesicles containing both endogenous and exogenous Sb2 was only ~0.33 of that found in vesicles containing only endogenous Sb2, indicating that for every one molecule/quantum of YSpH there are ~3 molecules of endogenous Sb2. A similar ratio was obtained when comparing Sb2 immunoreactivity/Atto signals from individual vesicles ( n =419) of untransfected astrocytes with those from dually laden vesicles ( n =499) of YSpH-expressing astrocytes ( Fig. 7c ); the additional Atto fluorescence of vesicles containing both endogenous and exogenous Sb2 was ~0.22 of that found in endogenous Sb2-only vesicles, which translates to ~5 endogenous Sb2 molecules for every YSpH molecule. 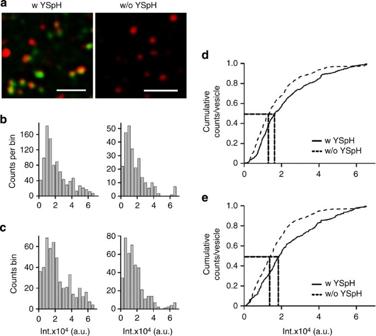Figure 7: Quantification of the ratio between the number of YSpH and endogenous Sb2 molecules in astrocytic vesicles. (a) Left fluorescent micrograph shows vesicles in cells transfected by YSpH and labelled by the Atto red dye (note that not all vesicles are labelled by both fluorophores), whereas the right panel shows vesicles in astrocytes labelled by the Atto dye only. Bar, 10 μm. (b,c) We obtained the distributions of Atto fluorescence intensity of Sb2 immunolabelled vesicles containing only endogenous Sb2 (w/o YSpH) and those that additionally contain exogenous Sb2 in form of YSpH (w YSpH). (b) Measurements were performed on vesicles within astrocytes expressing YSpH; some vesicles contained both endogenous Sb2 and YSpH (b, left) (n=958), while others were devoid of YSpH, expressing only endogenous Sb2 (b, right) (n=262). (d) The normalized cumulative counts of the Atto intensity inbshow significantly different distributions (D=0.134,P<0.001, Kolmogorov–Smirnov test). The vertical dotted lines drawn indicate the median value of 18,772 a.u. (with YSpH) and 14,115 a.u. (without YSpH) for Atto signals; horizontal dotted line indicates 50% of the total vesicle population. The difference between these two median values (4,657 a.u.) likely denotes the quantum fluorescence of exogenous Sb2, that is, YSpH, which was ~1/3 of that found in vesicles containing only endogenous Sb2. (c) Similar distribution as inb, only that we measured Atto fluorescence intensities of Sb2 immunolabelled vesicles in YSpH-expressing (c, left) (n=499) and in non-transfected astrocytes (c, right) (n=419), respectively. (e) The normalized cumulative counts of the Atto intensity incshow significantly different distributions (D=0.184,P<0.001, Kolmogorov–Smirnov test); the median values at 16,316 a.u. and 13,382 a.u. for Atto signals of w and w/o YSpH vesicles and the difference between these two median values (2,934 a.u.) suggests that exogenous Sb2 molecules represent ~1/5 of the number of endogenous Sb2 molecules; dotted lines as ind. Figure 7: Quantification of the ratio between the number of YSpH and endogenous Sb2 molecules in astrocytic vesicles. ( a ) Left fluorescent micrograph shows vesicles in cells transfected by YSpH and labelled by the Atto red dye (note that not all vesicles are labelled by both fluorophores), whereas the right panel shows vesicles in astrocytes labelled by the Atto dye only. Bar, 10 μm. ( b , c ) We obtained the distributions of Atto fluorescence intensity of Sb2 immunolabelled vesicles containing only endogenous Sb2 (w/o YSpH) and those that additionally contain exogenous Sb2 in form of YSpH (w YSpH). ( b ) Measurements were performed on vesicles within astrocytes expressing YSpH; some vesicles contained both endogenous Sb2 and YSpH ( b , left) ( n =958), while others were devoid of YSpH, expressing only endogenous Sb2 ( b , right) ( n =262). ( d ) The normalized cumulative counts of the Atto intensity in b show significantly different distributions (D=0.134, P< 0.001, Kolmogorov–Smirnov test). The vertical dotted lines drawn indicate the median value of 18,772 a.u. (with YSpH) and 14,115 a.u. (without YSpH) for Atto signals; horizontal dotted line indicates 50% of the total vesicle population. The difference between these two median values (4,657 a.u.) likely denotes the quantum fluorescence of exogenous Sb2, that is, YSpH, which was ~1/3 of that found in vesicles containing only endogenous Sb2. ( c ) Similar distribution as in b , only that we measured Atto fluorescence intensities of Sb2 immunolabelled vesicles in YSpH-expressing ( c , left) ( n =499) and in non-transfected astrocytes ( c , right) ( n =419), respectively. ( e ) The normalized cumulative counts of the Atto intensity in c show significantly different distributions (D=0.184, P< 0.001, Kolmogorov–Smirnov test); the median values at 16,316 a.u. and 13,382 a.u. for Atto signals of w and w/o YSpH vesicles and the difference between these two median values (2,934 a.u.) suggests that exogenous Sb2 molecules represent ~1/5 of the number of endogenous Sb2 molecules; dotted lines as in d . Full size image We have developed a new approach to label Sb2 with two different fluorescent tags and used super-resolution microscopy to visualize them in a living cell. To determine compartmentalization of proteins in vesicles of astrocytes [33] , we measured the length of Sb2 on a single vesicle in live cells in vitro . The lengths of Sb2 marked with YpH in the vesicle lumen and with a fluorescent protein (mCherry) or a dye conjugated with antibodies against Sb2 (Atto) present on the cytoplasmic site were 57 and 65 nm, respectively. These measurements are in accordance with theoretical values of ~54 nm and ~75–80 nm, respectively, given for the length of uncoiled Sb2, pHluorin, mCherry and antibodies [18] , [19] , [21] . However, unstructured Sb2 coils in the presence of syntaxin1 and/or the binary acceptor syntaxin1-SNAP25 complex [21] , [34] , an expected scenario in the cellular millieu, as in our experiments. As coiled Sb2 has three α-helices (I: 36–54 aa, II: 77–88 aa and III: 93–115 aa) [19] and the distance between two adjacent aa residues in the helical form of peptide or protein is smaller by ~0.15 nm than in an elongated form [35] , [36] , coiled Sb2 (containing total of 51 coiled aa) should be about ~8 nm shorter compared with an uncoiled version. Consequently, the theoretical expectations for the above measurements then would be ~47 nm and ~67–72 nm, values that can be readily observed in YpH-mCherry ( Fig. 3d ) and YpH-Atto ( Fig. 2f ) distributions around the peak measurements. Thus, it is likely that we have been observing a mixture of uncoiled and coiled Sb2; alternatively, the jitter in the measurement could be technical in nature (that is, already mentioned variability in fluorophore alignments with respect to the imaging plane). We measured the intensity of YpH and Atto from SIM images and classified YpH/Sb2 pairs into various categories based on the configurations or patterns of these fluorophores on astrocytic vesicles ( Fig. 2 ). The most common observed pattern ‘a’ likely represents a vesicle in which the number of Sb2 molecules is relatively low, as per comparable absolute intensities of YpH and Atto ( Fig. 2a , middle). The pattern ‘b’ whereby Atto fluorophore exhibited nearly three times higher fluorescence intensity than YpH intensity ( Fig. 2b , middle) could correspond to clustering of Sb2, as noted previously by an X-ray study [37] . Previous reports indicate that Sb2 undergoes dimerization specifically at the transmembrane domain [38] , [39] . YpH and Atto pattern ‘c’ ( Fig. 2c , middle) offers a dichotomous interpretation: (i) either the orientation of the Atto cluster is not parallel to the imaging plane or (ii) there may be two vesicles placed one over the other. The least common image observed pattern ‘d’ ( Fig. 2d , middle) was interpreted as Atto molecules present on two extremes of a vesicle circumference, while YpH is situated between two Atto puncta. Although it is tempting to use the distance between two peaks of Atto signal enveloping or flanking the YSpH signal to coarsely estimate the vesicle diameter, such measurements could cause errors associated with size and positioning of antibodies, and we have rather developed an alternative strategy to obtain the estimate of vesicular size in live astrocytes. Several approaches have been used to measure vesicle diameters in astrocytes [26] , [40] , [41] . Here we used a distinct approach based on Sb2 tagging in conjunction with dye filling of the vesicular lumen. After staining acidic organelles with LysoTracker, we obtained the apparent diameters of selected YSpH-laden vesicles as 305±4 nm in live astrocytes. This is likely a slight overestimation due to point-spread-function convolution, as seen in control experiments estimating the size of fluorescent beads of the known diameter. However, these measurements are in good agreement with measurements of vesicles tagged with Sb2 in live astrocytes investigated using evanescence wave microscopy; those vesicles showed an apparent diameter of ~312 nm (ref. 26 ). For our present measurements, only a subset of vesicles was interrogated due to the fact that a vesicle expressing a visible YSpH requires optimized pH in the vesicle lumen along with co-labelling with LysoTracker. Namely, LysoTracker stains mostly acidic compartments of astrocytes [25] , whereas YSpH becomes fluorescent once the fusion pore is open or by other mechanisms that lead to alkalinization. Some published reports provide information about the number of Sb2 proteins or SNARE complexes present on a vesicle membrane or number/ratio involved in the fusion of a vesicle membrane with the plasma membrane in neurons [5] , [42] , [43] , [44] , [45] , [46] . On the basis of changes in YSpH fluorescence, we estimated the number of YSpH molecules present in an astrocytic vesicle, as well as the number of YSpH molecules involved in fusion pore formation. The intensity patterns after application of ATP or NH 4 Cl were found to be different, indicating that the addition of ATP makes visible only some YSpH molecules due to dequenching mediated by partial and/or by restricted alkalinization of the vesicle lumen after opening of the narrow fusion pore. This is an intriguing finding as it may point out to an unappreciated mechanism for pH buffering of vesicular lumen and it should be explored in the near future. Alternatively, there could be a subpopulation of vesicles at the membrane that fuses when astrocytes are stimulated with ATP or vesicles are clustered, and only some have access to the extracellular alkaline medium or there may be a pH gradient in the vesicle lumen in case of comparable fluxes through pumps and the fusion pore. Nonetheless, addition of NH 4 Cl makes all the content of the vesicle lumen alkaline because ammonia in equilibrium with ammonium ions in solution diffuses across cell membranes and increases the pH [47] . Therefore, in single-vesicle experiments, pH change by ATP elicits fluorescence of a limited portion of all available luminal vesicle pH-sensitive fluorescent proteins or a limited number of vesicles in a cluster. The amplitude distribution plot for ATP shows a single mode ( Fig. 5c , middle). The amplitude distribution plot for NH 4 Cl with multiple modes ( Fig. 5c , right) signifies that after chemical alkalinization, all units of YSpH present in a vesicle lumen are fluorescent. If the modal peaks represent units or molecules, then these should represent simple integer multiples. Indeed, the mean of Gaussian distributions are equidistant with a value of 5 a.u., representing the fundamental quantal unit, which indicates the apparent number of YSpH units or molecules present in a single vesicle. The results show that there is at least one and not more than five YSpH (exogenous Sb2) units or molecules present on an astrocytic vesicle ( Fig. 5d ). On the basis of a single-mode distribution during ATP stimulation, it is most likely that only one YSpH molecule is involved in initial fusion pore formation during the merger between vesicle and plasma membranes in astrocytes. Indeed, these measurements were limited to kiss-and-run events as full fusion would cause dissipation of YSpH signal in the plasma membrane as vesicular membrane collapses to and dilutes its content within the plasma membrane [26] . The time-dependent intensity profile for each fluorescent punctum, present in a cell after stimulation with ATP and NH 4 Cl, demonstrated three different types of events ( Fig. 5b ). The most abundant event type in an astrocyte is an NH 4 Cl-elicited increase in YSpH fluorescence preceded by the failure of ATP stimulation to evoke such a response. ATP influences two types of events: one shows a step increase in fluorescent intensity after ATP that is further enhanced by the addition of NH 4 Cl and another type of event also shows a step increase after ATP but, after approximately 1 min, it returns to the initial intensity, which then increases with the addition of NH 4 Cl. This rare event may be due to the fact that a secretory vesicle situated close to the plasma membrane can form a stable fusion pore [48] . We also obtained a comparable estimated number of YSpH molecules using photobleaching of alkalinized YSpH-laden vesicles. Thus, the estimated numbers of exogenous Sb2 molecules per vesicle in live astrocytes ( Figs 5 and 6 ) appear similar using two approaches (ATP or NH 4 Cl-mediated YSpH increase and photobleaching of NH 4 Cl-alkalinized YSpH-laden vesicles) that cross-check each other (that is, three to five exogenous Sb2 molecules). Furthermore, we determined the ratio of endogenous Sb2 to YSpH molecules per vesicle, leading us to conclude that individual astrocytic vesicles contain ~15–25 molecules of Sb2, which is ~3–5 times smaller amount than the previously reported value of ~70 copies of this SNARE protein per individual neuronal, that is, synaptic vesicle [42] . In summary, the results provide a new insight into the nano architecture of Sb2 on an astrocytic vesicle, which is playing a role in vesicle fusion and gliotransmitter release from astrocytes. Cell culture Cortical astrocytes from 3-day-old female rats used in the experiments were isolated as described [49] . The care for experimental animals and the euthanization of animals were carried out in strict accordance with the following ethical codes and directives: The International Guiding Principles for Biomedical Research Involving Animals developed by the Council for International Organizations of Medical Sciences and the Directive on Conditions for Issue of License for Animal Experiments for Scientific Research Purposes (Official Gazette of the Republic of Slovenia 40/85, 22/87, 43/07). The protocol for the euthanization of the animals used in our study was approved by the Veterinary Administration of the Ministry for Agriculture and the Environment of the Republic of Slovenia (permit No: 34401-29/2009/2), issued on 22.4.2009; procedures were also in strict accordance with the National Institutes of Health Guide for Care and Use of Laboratory Animals and were approved by the University of Alabama, Birmingham Institutional Animal Care and Use Committee. Astrocytes were plated on poly- L -lysine-coated coverslips and cultured with Dulbecco's modified Eagle medium (DMEM, high glucose content: 4,500 mg l −1 ) supplemented with 10% fetal bovine serum (FBS), 1 mM sodium pyruvate, 2 mM L -glutamine and 25 μg ml −1 penicillin-streptomycin antibiotics in 95% air and 5% CO 2 atmosphere at 37 °C. Unless stated otherwise, all chemicals were obtained from Merck (Darmstadt, Germany) and Sigma (Diesenhofen, Germany). For experiments in Supplementary Fig. 1 , cultured purified primary rat astrocytes were obtained from visual cortices of 1- to 2-day-old Sprague–Dawley rats [8] . Plasmid construction Green superecliptic synaptopHluorin (GSpH), a fluorescent Sb2 derivative, is a fusion protein chimera consisting of mouse Sb2 and modified EGFP, pHluorin, fused to Sb2 C terminus inside the vesicle lumen. On the basis of known amino acids contributing to chromophore pockets of EGFP versus EYFP [50] , [51] , we introduced mutations to GSpH to generate its yellow-shifted emission variant. This YSpH was constructed by polymerase chain reaction (PCR) mutagenesis using the original GSpH plasmid generously provided by Dr James E. Rothman (Yale University, New Haven, CT) [17] , [52] . Four primers were utilized containing mutations as well as 15-bp overlapping sequences for use with the InFusion 2 system (Clontech Laboratories, Mountainview, CA). PCR for both vector and insert fragments (listed below) was performed on a GSpH template introducing the desired mutations, and the resulting fragments were rejoined with InFusion 2 enzyme and buffers according to the manufacturer’s instructions. The resulting plasmid ( PYSpH ) was sequenced and expressed in rat primary astrocyte culture using cytomegalovirus immediate early promoter contained in plasmid ( Supplementary Fig. 1 for details). Vector primers Fwd 5′-TACCAGACAACCATTACCTGTTTTACACTTCTACTC-3′ Rev 5′-AGCATTGCAGACCATAGCCGAAAGTAG-3′ Insert primers Fwd 5′-ATGGTCTGCAATGCTTTGCCAGATAC-3′ Rev 5′-AGTGTAAAACAGGTAATGGTTGTCTG-3′ Using the InFusion 2 subcloning system, we made two additional plasmids, one encoding YSpH additionally tagged by the red fluorescent protein mCherry on the cytoplasmic vesicle site ( PmCherry-YSpH ) and the other ( PYSpH-7aa-mCherry ) encoding the chimeric protein YSpH-7aa-mCherry in which mCherry was appended to the C terminus of YSpH via a 7-aa linker (see Supplementary Fig. 2 for plasmid maps). PCR for the vectors was performed on the YSpH template, while the PCR for the mCherry insert fragments was performed on the pcDNA3.1/VChR1-mCherry plasmid, kindly provided by Dr Karl Deisseroth (Stanford University, Stanford, CA) [4] . The DNA sequence (5′-tcaggtctacgatctagagct-3′) of the polypeptide linker (SGLRSRA), as we previously used [5] , was introduced by primer overhangs. Plasmid constructs were checked by restriction enzyme digestion and sequencing before expression in primary astrocyte culture. Primers used in subcloning are listed below. mCherry-YSpH Vector Primers: Fwd 5′-TGTACAAGTCGGCTACCGCTGCCACCGTC-3′ Rev 5′-CTTGCTCACCATGGTGGCACGCGTGAATTC-3′ mCherry-YSpH Insert Primers: Fwd 5′-ACCATGGTGAGCAAGGGCGAGGAG-3′ Rev 5′-TAGCCGACTTGTACAGCTCGTCCATG-3′ YSpH-7aa-mCherry Vector Primers: Fwd 5′-TAATCTAGAGTCGACCCGGGCGGCCGCTTCCCTTTAG-3′ Rev 5′-AGATCGTAGACCTGAACCGGTTTTGTATAGTTCATCCATGCCATG-3′ YSpH-7aa-mCherry Insert Primers: Fwd 5′-TCAGGTCTACGATCTAGAGCTGTGAGCAAGGGCGAG-3′ Rev 5′-GTCGACTCTAGATTACTTGTACAGCTCGTCCATG-3′. Plasmid DNA transfection Astrocytes were transfected with 1–2 μg of pDNA [6] , [7] using FuGENE 6 transfecting reagent (Roche, Mannheim, Germany) and the culture medium as above (without FBS). UltroserG (3%; Life Technologies) was added after an incubation period of 3 h at 37 °C, and the cells were then incubated overnight. The transfected astrocytes were examined or immunolabelled after at least 24 h incubation. In a subset of experiments ( Supplementary Fig. 1 ), astrocytes were transfected with plasmids using TransIT 293 transfection reagent (Mirus Bio, Madison, WI) [8] . Immunocytochemistry The transfected astrocytes were washed with phosphate-buffered saline (PBS), fixed in 4% formaldehyde (Thermo Scientific, USA) in PBS for 15 min and incubated in 0.1% Triton X-100 for 10 min at room temperature. Nonspecific background staining was reduced by blocking buffer containing 3% bovine serum albumin (BSA) and 10% goat serum in PBS (37 °C, 1 h). We used mouse polyclonal primary antibody raised against a synthetic peptide corresponding to amino acids 1–18 of Sb2 (1:500; Abcam, Cat. No. ab3347). Astrocytes were incubated with an anti-Sb2 antibody diluted in 3% BSA in PBS for 2 h at 37 °C or overnight at 4 °C. The cells were then stained with secondary antibodies against mouse IgG conjugated to Atto 594 (1:100; Sigma Aldrich) at 37 °C for 45 min. The cells were again rinsed four times with PBS and mounted on glass slides using SlowFade Gold antifade reagent (Invitrogen, Eugene, OR). Optical imaging CLSM: Cells were examined with an inverted Zeiss LSM 510 META microscope (Germany) with a 63 × /1.4 Oil DIC objective, He/Ne and argon lasers. YSpH was excited by a 488 nm line. The light emitted was collected through a band-pass filter (505–530 nm). SIM: The detailed architecture of astrocytic vesicles was examined using a Zeiss ELYRA PS.1 super-resolution microscope (Germany) equipped with five different grating frequencies for SIM for optimal matching of the illumination pattern to the laser wavelength and objective lens. The cells were scanned using a Plan-Apochromat 63 × /1.4 Oil DIC M27 objective and HBO X-Cite 120 lamp. Cells were illuminated with laser lines (561 and 488 nm). Sixteen-bit images were acquired with an EMCCD camera (Andor iXon 885) with variable exposure. The diameter of standard beads used in the intensity analysis was 200 nm (Zeiss, Germany). Additional details for the imaging used in a subset of Supplementary Fig. 1 can be found in Supplementary Methods . Single-vesicle pHluorin experiments Astrocytes expressing YSpH were scanned using an LSM 510 META microscope. The cells were kept in 200 μl of extracellular solution for live imaging, consisting of (in mM) 130 NaCl, 5 KCl, 2 CaCl 2 , 1 MgCl 2 , 10 D -glucose, 10 N -2-hydroxyethylpiperazine- N ′-2-ethanesulphonic acid (HEPES), pH 7.2 and ~300 mOsm kg −1 . To increase the free concentration of calcium ions ([Ca 2+ ] i ) in the cytoplasm, astrocytes were stimulated with 0.1 mM ATP. Extracellular solution containing 45 mM NH 4 Cl was used for the vesicle alkalinization. A time-lapse imaging series of 200 frames (1 frame s −1 ) was acquired. During acquisition, we applied ATP and NH 4 Cl at 30 s and 120 s, respectively, and left until the end of experiments. In photobleaching experiments, a time-lapse imaging series of 300 frames (1 frame s −1 ) was acquired. During acquisition, we applied NH 4 Cl at 10 s and increased the laser power by factor of 2–3 after 50 s and both left until the end of experiments. To stain the vesicle lumen for measurement of vesicle diameter, transfected astrocytes were incubated with 100 nM LysoTracker Red DND-99 (Molecular Probes) at 37 °C for 5 min. Image and data analysis To quantitatively analyse large collections of images, we developed a custom tool ColocAna (Celica, Slovenia) using Matlab (Mathworks, Natick, MA). The colocalization of Atto and YpH was analyzed, as reported (Kreft et al ., [33] ), by using ColocAna software that counts red, green and colocalized pixels. The colocalization was calculated for all pixels above the threshold, which was set at 20% of maximum green and red fluorescence intensity and was expressed as the percentage of colocalized green pixels. The distance between two fluorophores is measured using a ZEN lite software (Carl Zeiss) by drawing a line profile on two different fluorophores in each of Atto-YpH and mCherry-YpH pairs. To measure the diameter of astrocytic vesicles, we calculated the average values of FWHM of the line profile drawn for a LysoTracker-stained vesicle [53] ; for better precision, we drew crosshair line profiles in the x and y directions of the 2D plane of each punctum. Levenberg-Marquadt X 2 minimization for nonlinear least-square fitting was performed in OriginLab Pro. 8 software to fit the Gaussian curve on the histograms. The intensity analysis for the pHluorin experiments was done with ImageJ 1.35j software (National Institutes of Health, USA) by selecting square regions of interest (1.33 × 1.33 μm 2 ) overlaid on each fluorescent punctum, and thereby mean intensities were estimated using the intensity versus time monitor plugin. Statistical analysis The values for the Gaussian fit are given as mean±s.e.m. Statistical significance of the data was analyzed in the SigmaPlot version 11 software. P -values <0.05 were considered to be statistically significant. How to cite this article: Singh, P. et al . Single-vesicle architecture of synaptobrevin2 in astrocytes. Nat. Commun. 5:3780 doi: 10.1038/ncomms4780 (2014).